Distinct charge dynamics in battery electrodes revealed byin situandoperandosoft X-ray spectroscopy Developing high-performance batteries relies on material breakthroughs. During the past few years, various in situ characterization tools have been developed and have become indispensible in studying and the eventual optimization of battery materials. However, soft X-ray spectroscopy, one of the most sensitive probes of electronic states, has been mainly limited to ex situ experiments for battery research. Here we achieve in situ and operando soft X-ray absorption spectroscopy of lithium-ion battery cathodes. Taking advantage of the elemental, chemical and surface sensitivities of soft X-rays, we discover distinct lithium-ion and electron dynamics in Li(Co 1/3 Ni 1/3 Mn 1/3 )O 2 and LiFePO 4 cathodes in polymer electrolytes. The contrast between the two systems and the relaxation effect in LiFePO 4 is attributed to a phase transformation mechanism, and the mesoscale morphology and charge conductivity of the electrodes. These discoveries demonstrate feasibility and power of in situ soft X-ray spectroscopy for studying integrated and dynamic effects in batteries. Improving energy storage technology has become a critical and formidable challenge for modern sustainable energy applications, especially for electric vehicles. Lithium-ion battery (LIB) technology provides a high-efficiency solution for energy storage. However, significant improvements in cost, safety, capacity and power density are needed for current LIBs to meet the requirements for transportation applications [1] . A practical LIB electrode is a complex system consisting of active materials, electrolyte, binder, additives and current collectors. LIBs operate with ion and electron migration through such integrated matrix, leading to evolving chemical and physical states in electrodes throughout electrochemical cycles. Although ex situ techniques have provided much valuable information for understanding individual components in equilibrium states, the dynamics of LIB, as one integrated multicomponent system, can only be characterized through in situ experiments. Tremendous efforts have been made to develop various in situ techniques based on hard X-ray [2] , electron microscopy [3] , neutron scattering [4] and nuclear magnetic resonance [5] for battery research. In particular, because of its penetration depth, hard X-ray techniques such as diffraction [2] , [6] and absorption spectroscopy [2] , [7] have received early and wide use for in situ studies of batteries. Compared with hard X-ray and other techniques, soft X-ray spectroscopy [7] , [8] , [9] , [10] is a more direct and efficient experimental probe of the electronic states near the Fermi level. In battery materials, these key electronic states in the vicinity of Fermi level fundamentally regulate the properties pertaining to battery performance [9] , such as electron conductivity [11] , ion diffusion [12] , open-circuit voltage [13] , safety [14] , structural stability [15] and phase transformation [16] . In particular, for transition-metal (TM) oxide-based cathodes, TM- 3d and anion- p states can be directly detected using soft X-ray absorption spectroscopy (sXAS) through dipole-allowed transitions [7] , [8] , [9] , [10] , [17] . However, the short penetration depth of soft X-rays requires ultrahigh vacuum or high vacuum environments for sXAS experiments. Several recent in situ studies using soft X-ray absorption [18] , photoemission spectroscopies [19] and microscopy [20] have generated important results on specially designed model electrochemical cells; however, in situ sXAS of a real LIB cell remains challenging because of the complexity of LIBs. In this work, we have developed an in situ system for sXAS studies of LIBs. Two different electrode systems are deliberately selected and compared. The surface sensitivity of soft X-ray techniques is utilized for position-dependent studies of charge transportation during battery operations. Combining battery fabrication, morphology characterization, and in situ and ex situ sXAS techniques, we are able to unveil the charge dynamics in battery electrodes that are regulated by charge transport, mesoscale morphology and phase transformation. Additionally, the contrast between different electrode systems and the comparison between in situ and ex situ results provide soft X-ray fingerprints of metastable phases during the electrochemical process. In situ and operando soft X-ray system for LIB studies To overcome the technical difficulties of sXAS experiments because of both the shallow penetration depth and ultrahigh vacuum requirements, we modified the current collector at the initial stage of cell fabrication and utilized polymer electrolyte. The specially designed setup is depicted in Fig. 1 . The current collector on top is an aluminium foil with detection windows of 50-μm diameter holes drilled with a programmable, high-power and high-precision laser system ( Fig. 1b ). Owing to the inherent elemental sensitivity of sXAS [10] , signal from Al foil that is exposed to X-rays does not contribute any feature to the spectra of electrodes collected through the detection holes. Several designs of the detection windows with different sizes, shapes and patterns have been tested. As demonstrated in the results below, the design implemented here allows direct soft X-ray measurements on the electrode materials, meanwhile maintaining normal electrochemical operation. 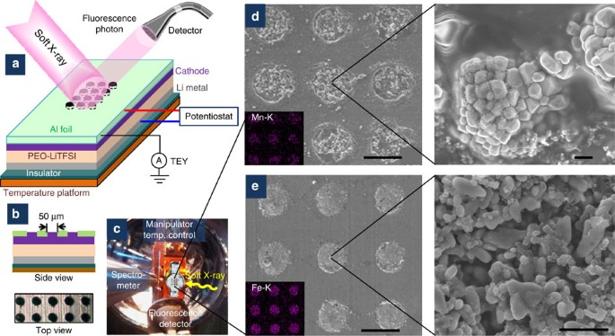Figure 1:In situbattery cell and electrode mesoscale morphology. (a,b) The schematic depiction of experimental setup of thein situcell for simultaneous cycling and X-ray spectroscopic measurement. An array of holes with 50 μm diameter is drilled with high-precision laser on the current collector. The incident soft X-ray beam and excited fluorescence photon pass through the array of holes on the current collector. (c) A photo of thein situsoft X-ray setup for studying LIBs. (d,e) SEM and energy dispersive X-ray spectroscopy images of the top surfaces of thein situcells after the cathode layers formed with the slurry process for NMC (d) and LFP (e) electrodes. The scale bars are 100 μm in the left panels and 1 μm in the right panels, respectively. Images shown here are after one electrochemical cycle, and we did not observe morphological difference before and after the cycling. NMC forms large secondary particles that are composed of agglomerated primary smaller particles. Electrolyte matrix forms microdomains in NMC (d), whereas it is superficially distributed on LFP nanoparticles (e). Figure 1: In situ battery cell and electrode mesoscale morphology. ( a , b ) The schematic depiction of experimental setup of the in situ cell for simultaneous cycling and X-ray spectroscopic measurement. An array of holes with 50 μm diameter is drilled with high-precision laser on the current collector. The incident soft X-ray beam and excited fluorescence photon pass through the array of holes on the current collector. ( c ) A photo of the in situ soft X-ray setup for studying LIBs. ( d , e ) SEM and energy dispersive X-ray spectroscopy images of the top surfaces of the in situ cells after the cathode layers formed with the slurry process for NMC ( d ) and LFP ( e ) electrodes. The scale bars are 100 μm in the left panels and 1 μm in the right panels, respectively. Images shown here are after one electrochemical cycle, and we did not observe morphological difference before and after the cycling. NMC forms large secondary particles that are composed of agglomerated primary smaller particles. Electrolyte matrix forms microdomains in NMC ( d ), whereas it is superficially distributed on LFP nanoparticles ( e ). Full size image We applied poly(ethylene oxide) (PEO)-lithium bis(trifluoromethanesulphonyl)imide (LiTFSI) as the solid-state electrolyte. The electrodes are cast by mixing the active materials with acetylene black (AB) conductive additive, PEO and LiTFSI salt (see Methods). The assembled battery cell was mounted on a plate with electric contacts for electrochemical cycling and temperature control ( Fig. 1c ). In order to avoid radiation-damage issues with polymer electrolyte, both the X-ray flux and beam size are carefully tested and controlled with a dedicated refocusing mirror system (see Methods). Although the original purpose of using polymer electrolyte is to simplify the technical design, our results show interesting charge transportation behaviour related to polymer electrolyte, indicating that this setup may also be applied for solid-state electrolyte studies. We selected two cathode materials with different types of electrochemical behaviours, LiCo 1/3 Ni 1/3 Mn 1/3 O 2 (NMC) [21] and LiFePO 4 (LFP) [22] . NMC is a known layered material with solid-solution type of Li-ion diffusion [21] . LFP with standard particle size shows dominating two-phase transformation mechanism during the (de)lithiation process [22] . Both materials are extensively investigated by ex situ soft X-ray techniques [7] , [8] , [23] , [24] , allowing us to compare our in situ observations with ex situ results. From our comprehensive tests, results from seven cells are summarized herein ( Supplementary Table S1 ). Scanning electron microscopy (SEM) and energy dispersive X-ray spectroscopy confirm that the cathode materials are confined inside the holes with negligible spill ( Fig. 1d,e , Supplementary Fig. S1 ). Additionally, the SEM images show that the NMC and LFP electrodes display very different mesoscale morphology. The NMC used in this study forms the so-called secondary particles with micro-size domains of electrolyte ( Fig. 1d ) [25] . LFP electrode shows well-separated nanoparticles with superficially distributed electrolyte ( Fig. 1e ). The large NMC secondary particle in Fig. 1d implies reduced surface area. We measured the surface area of NMC and LFP materials by using a surface area analyser through the standard Brunauer–Emmett–Teller (BET) method. The specific area of NMC (0.171±0.007 m 2 g −1 ) is about 75 times smaller than that of the LFP (12.823±0.011 m 2 g −1 ). Operando sXAS demonstrated in NCM electrodes We first demonstrate the success of our technical approach on in situ and operando sXAS experiments of LIBs. 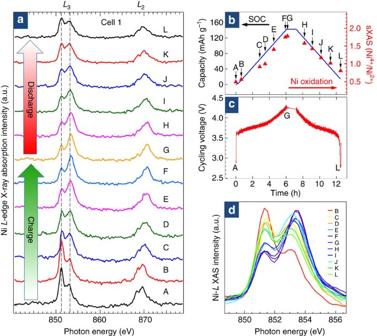Figure 2:OperandosXAS of a NMC/PEO-LiTFSI/Li battery cell. (a) NiL-edge sXAS TFY spectra of NMC cathode in Cell 1. Data were collected simultaneously with electrochemical cycling with C/5 rate. Spectra are taken at different SOC levels, denoted as A–L. Intensity ratio of the furtherL3splits (dotted lines) fingerprints the oxidation states of Ni. (b) Ni oxidation states (red triangle) obtained from spectra shown in (a) plotted together with specific capacity cycling curve (blue line) of Cell 1 from electrochemical measurements. The sXAS results follow the SOC in electrochemical cycling in real time. (c) Cycling voltage versus time of Cell 1. The potential changes between 2.8 and 4.2 V throughout the cycling period, indicating solid-solution type phase transformation in NMC. (d) Stacked Ni-L3spectra show no isosbestic point, consistent with (c) on the solid-solution type of phase transformation. Figure 2 shows the in situ sXAS results of a NMC/PEO-LiTFSI/Li cell (Cell 1) during a full cycle, starting from as-prepared discharged state. Total fluorescence yield (TFY) signal of Ni L -edge, with about 100 nm probe depth, was collected in real-time when the cell was electrochemically cycled ( Fig. 2a ). For all 3d TM elements, sXAS directly measures the unoccupied TM- 3d states through dipole-allowed 2p-to-3d transitions [10] . Ni L -edge XAS corresponds to the excitation of Ni 2p core electrons to the empty 3d orbitals. The overall spectra lineshape consists of features in two regions, L 3 around 852 eV and L 2 around 870 eV, resulting from the core-hole spin-orbital-coupling split. Further, high-resolution sXAS spectra resolve the fine splittings of the features because of the multiplet effect from Ni 2p-3d interactions and crystal field effect from local ligand environment [10] . The intensity ratio of the double-peak features in the Ni- L 3 region, at 851.2 and 853.1 eV (dotted lines), fingerprints the oxidation states of Ni, which changes from Ni 2+ to Ni 4+ during charge process (A-F), and vice versa during discharge (G-L) [7] . Total electron yield (TEY) signal of sXAS ( Supplementary Fig. S2 ), with about 10-nm probe depth, is consistent with TFY in the trend of lineshape change but shows lower Ni oxidization states, especially when fully charged (Spectrum G). Except for the higher resolution of our spectra, both the Ni- L spectral lineshape evolution and the Ni oxidation state gradient are consistent with ex situ results of NMC [7] and other Ni-contained cathodes [26] , [27] , [28] , [29] . Additionally, TFY and TEY of sXAS of Mn and Co L -edges ( Supplementary Fig. S2a–c ) confirm that oxidation states of Mn and Co remain unchanged with cycling voltage <4.2 V. The reproducibility of in situ sXAS results is verified by measuring an identical cell (Cell 2) from charged state ( Supplementary Fig. S3 ). Figure 2: Operando sXAS of a NMC/PEO-LiTFSI/Li battery cell. ( a ) Ni L -edge sXAS TFY spectra of NMC cathode in Cell 1. Data were collected simultaneously with electrochemical cycling with C/5 rate. Spectra are taken at different SOC levels, denoted as A–L. Intensity ratio of the further L 3 splits (dotted lines) fingerprints the oxidation states of Ni. ( b ) Ni oxidation states (red triangle) obtained from spectra shown in ( a ) plotted together with specific capacity cycling curve (blue line) of Cell 1 from electrochemical measurements. The sXAS results follow the SOC in electrochemical cycling in real time. ( c ) Cycling voltage versus time of Cell 1. The potential changes between 2.8 and 4.2 V throughout the cycling period, indicating solid-solution type phase transformation in NMC. ( d ) Stacked Ni- L 3 spectra show no isosbestic point, consistent with ( c ) on the solid-solution type of phase transformation. Full size image Red triangles in Fig. 2b show the evolution of Ni oxidation state derived by ratio of the peak intensities at 853.1 and 851.2 eV in Fig. 2a . This sXAS evolution follows the electrochemical state-of-charge (SOC) (blue line in Fig. 2b ) throughout the battery operation. Therefore, our in situ sXAS does provide elemental sensitive fingerprints of the electrochemical process in NMC/PEO-LiTFSI/Li cells in real time. In situ sXAS of LFP electrodes without relaxation On the contrary, the LFP electrodes in LFP/PEO-LiTFSI/Li battery cells, which are prepared and cycled in the same way as that for NMC/PEO-LiTFSI/Li cells, exhibit no real-time response of in situ sXAS to electrochemical cycling. First of all, previous ex situ studies of LFP systems [8] , [23] , [24] show high sensitivity of Fe- L sXAS to the SOC levels in LFP ( Supplementary Fig. S4 ). In particular, the intensity ratio of the Fe -L 3 features at 706 and 708 eV fingerprints the different Fe oxidation states in charged (Fe 3+ ) and discharged (Fe 2+ ) LFP electrodes. The high sensitivity of Fe L- edge sXAS to the (de)lithiation level could allow even quantitative definition of the SOC levels in the electrodes [7] . Surprisingly, the in situ TEY and TFY sXAS spectra of Fe L -edge at different charging stages do not display any response to the electrochemical process from discharged to charged states ( Fig. 3a–d ). Within the probe depth of soft X-ray, the unchanged in situ spectra indicate that Fe remains dominatingly at the initial discharged (Fe 2+ ) state, even though the overall LFP electrode is electrochemically charged ( Fig. 3a–d ). 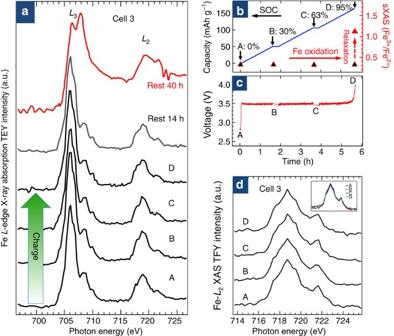Figure 3: Strong relaxation effect ofin situsXAS. (a) FeL-edge sXAS TEY spectra of the LFP cathode in Cell 3 at different electrochemical cycling stages labelled as A–D in the initial charge cycle and after 14 and 40 h of relaxation. The lineshape atL3around 706 eV andL2around 719 eV again fingerprints the oxidation state of Fe in LFP, which does not show any change without long relaxation. (b) Specific capacity curve (blue line) ofin situCell 3, plotted together with the Fe oxidation state derived fromin situsXAS before (black triangle) and after (red triangle) relaxation. (c) Cycling voltage versus time of Cell 3 show the typical plateau at about 3.4 V for LFP electrodes, indicating the two-phase transformation. (d) Fe-L2sXAS TFY spectra of the same LFP cathode. Inset shows overlapping spectra A-D, no change is observed without relaxation. Figure 3: Strong relaxation effect of in situ sXAS. ( a ) Fe L -edge sXAS TEY spectra of the LFP cathode in Cell 3 at different electrochemical cycling stages labelled as A–D in the initial charge cycle and after 14 and 40 h of relaxation. The lineshape at L 3 around 706 eV and L 2 around 719 eV again fingerprints the oxidation state of Fe in LFP, which does not show any change without long relaxation. ( b ) Specific capacity curve (blue line) of in situ Cell 3, plotted together with the Fe oxidation state derived from in situ sXAS before (black triangle) and after (red triangle) relaxation. ( c ) Cycling voltage versus time of Cell 3 show the typical plateau at about 3.4 V for LFP electrodes, indicating the two-phase transformation. ( d ) Fe- L 2 sXAS TFY spectra of the same LFP cathode. Inset shows overlapping spectra A-D, no change is observed without relaxation. Full size image Strong relaxation effect in LFP electrodes In order to rule out the possibility that the material inside the detection-hole area of the LFP cell (Cell 3) is inactive, we left Cell 3 at the charged status under open-circuit condition at room temperature. As shown in Fig. 3a , after about 40 h of relaxation with no further charging, the spectrum displays strong character of the charged (Fe 3+ ) state. This testifies that the material enclosed in the detection holes of the in situ cell is active but responds extremely slow to the electrochemical process. Based on the observation of the long relaxation effect of LFP electrodes in Cell 3, we are able to achieve a set of evolving in situ Fe- L sXAS spectra by maintaining the temperature at 75 °C and relaxing it for about 4 h at each stage ( Fig. 4a ). Additionally, we fabricated another cell with higher concentration of electrolyte/binder in the cathode (Cell 5 in Supplementary Table S1 ). Cell 5 still exhibits relaxation behaviour; however, the relaxation time is significantly shortened. After resting for only 26 h at room temperature, the spectrum shows almost fully charged (Fe 3+ ) state ( Supplementary Fig. S5 ). This change is much faster and stronger than that of Cell 3 after 40 h of relaxation ( Fig. 3a ). As the ion conductivity increases with the concentration and temperature of polymer electrolyte, both the temperature and electrolyte-concentration dependence indicate that the relaxation time shortens greatly with high ion conductivity. 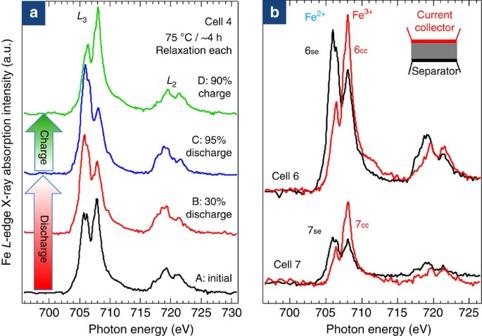Figure 4:In situandex situsXAS of LFP/PEO-LiTFSI/Li battery cells. (a)In situFeL-edge sXAS of LFP in Cell 4. The cell was kept at 75 °C during both the cycling and the 4-h relaxation before collecting the spectra. Fe oxidation state evolves with electrochemical cycling. (b)Ex situFeL-edge sXAS of cathodes in Cells 6 and 7, prepared with low and high electrolyte concentrations (Supplementary Table S1). Both cells were electrochemically charged but without long relaxation. Electrochemically charged (Fe3+) state obviously starts from the region adjacent to current collector (red). SOC gradient is stronger in Cell 6 with relatively low electrolyte concentration. Figure 4: In situ and ex situ sXAS of LFP/PEO-LiTFSI/Li battery cells. ( a ) In situ Fe L -edge sXAS of LFP in Cell 4. The cell was kept at 75 °C during both the cycling and the 4-h relaxation before collecting the spectra. Fe oxidation state evolves with electrochemical cycling. ( b ) Ex situ Fe L -edge sXAS of cathodes in Cells 6 and 7, prepared with low and high electrolyte concentrations ( Supplementary Table S1 ). Both cells were electrochemically charged but without long relaxation. Electrochemically charged (Fe 3+ ) state obviously starts from the region adjacent to current collector (red). SOC gradient is stronger in Cell 6 with relatively low electrolyte concentration. Full size image Position-dependent ex situ sXAS of LFP electrodes To further understand the origin of the retarded response of in situ sXAS to the electrochemical process in LFP electrodes, we performed ex situ sXAS experiments on the two opposite sides—that is, facing the separator and the current collector—of two LFP electrodes in Cells 6 and 7 ( Fig. 4b ). Cell 6(7) is prepared in the same way as the in situ Cell 3(5) with no holes in current collector. Cell 6 has lower electrolyte concentration in its LFP electrode than that in Cell 7 ( Supplementary Table S1 ). After the initial charge, the cells were immediately disassembled in an Ar glove box and transferred to the sXAS experimental chamber within 2 h, without any rinsing and air exposure. In this case, the ex situ sXAS measures the ‘frozen’ SOC in the electrodes before long relaxation. Strikingly, for both cells, the Fe- L sXAS collected on the side towards current collectors is consistent with the electrochemically charged state, displaying Fe 3+ (charged) spectra. The surfaces of electrodes towards separators, however, varied very little from the original Fe 2+ state for Cell 6. For Cell 7 with higher electrolyte concentration, the contrast between the two sides of the electrode becomes less; however, it is still obvious. The surface facing separator displays about half way towards charged Fe 3+ state in Cell 7 ( Fig. 4b ). Previously, we have demonstrated that sXAS is a sensitive probe to measure the subtle deviation from two-phase transformation in the LFP system [8] . The deviation manifests itself through deteriorating a perfectly defined isosbestic point in high-resolution spectra. In a solid-solution phase transformation system—for example, NMC—no isosbestic point could be defined in spectroscopy ( Fig. 2d , Supplementary Fig. S5 ). Cycling LFP is typically considered a two-phase process with standard particle size [22] . However, the finite deviation from two-phase process in LFP could be critical for understanding its facile ion diffusion, which likely stems from evolving metastable phases [30] , [31] . The in situ sXAS results of LFP ( Fig. 5b , bottom) display only a roughly defined isosbestic point, contrasting the perfect point defined in chemically delithiated LFP systems ( Supplementary Fig. S4b ). As an overall isosbestic point could still be defined, the in situ sXAS spectra indicate that the system remains dominatingly two-phase; however, the deviation from two-phase is obviously stronger than that in electrochemically prepared samples that have rested for a week before sXAS experiments [8] . Therefore, the in situ data provide additional experimental evidence for the existence of a metastable phase that deviates from two-phase transformation and evolves with time in LFP systems. 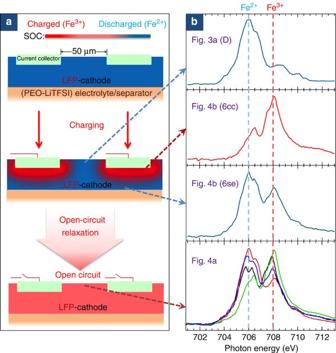Figure 5: Charge dynamics in LFP electrodes. (a) Schematic of the charging process of LFP electrodes revealed by the combinedin situandex situsXAS results. The SOC evolves from middle to bottom panels during open-circuit relaxation process, with the same averaged SOC value. (b) Summary of the key sXAS spectra that reveals the SOC configurations during the charging process of LFP electrodes. Bottom panel shows stacked Fe-L3sXAS spectra inFig. 4a. A roughly defined isosbestic point indicates the dominating two-phase transformation, but with finite deviation, in LFP electrodes (see text). Figure 5: Charge dynamics in LFP electrodes. ( a ) Schematic of the charging process of LFP electrodes revealed by the combined in situ and ex situ sXAS results. The SOC evolves from middle to bottom panels during open-circuit relaxation process, with the same averaged SOC value. ( b ) Summary of the key sXAS spectra that reveals the SOC configurations during the charging process of LFP electrodes. Bottom panel shows stacked Fe- L 3 sXAS spectra in Fig. 4a . A roughly defined isosbestic point indicates the dominating two-phase transformation, but with finite deviation, in LFP electrodes (see text). Full size image The schematic of our self-consistent findings on the charge dynamics in LFP electrodes is summarized in Fig. 5 . Immediately after an as-prepared LFP (Fe 2+ ) electrode is electrochemically charged (mid panel), the in situ sXAS measured through 50-μm detection holes remains unchanged (Fe 2+ ) ( Fig. 3 and Supplementary Fig. S3 , spectra before relaxation). Consistently, the ‘locked’ SOC detected using ex situ sXAS shows very small change on the electrode surface facing separator, whereas the surface adjacent to the current collector exhibits the electrochemically charged SOC (Fe 3+ ) state ( Fig. 4b ). After long time relaxation, the SOC in the electrode reaches overall uniformity, and in situ sXAS eventually shows responsive evolution to the averaged electrochemical status ( Fig. 3 and Supplementary Fig. S3 , after relaxation). Therefore, taking advantage of the surface sensitivity of sXAS, we are able to differentiate the evolution of SOC in the middle and bottom panels of Fig. 5a . As the relaxation takes place under open-circuit condition, the SOC distribution evolves with time but the averaged value remains the same. Therefore, such dynamic effect is invisible with other in situ techniques that take the whole (averaged) electrode into account. The discovery of the relaxation effect of SOC distribution in LFP electrode is significant. First, the SOC gradient does not simply depend on the side of electrodes but on the distance to current collector. The change of SOC is initiated in the region adjacent to current collector ( Fig. 5a ), indicating that the Li-ion diffusion across the electrode is facile enough with the PEO polymer electrolyte at 75 °C. This is a big surprise because, in conventional wisdom, ion diffusion is typically considered the rate-limiting process even with liquid electrolyte. Second, the open-circuit relaxation is driven by Li-ion diffusion. This is evidenced by the strong temperature and concentration dependence of relaxation time ( Fig. 4a and Supplementary Fig. S5 ). Previous ex situ sXAS [8] and soft X-ray microscopic [32] results show small or no gradient of SOC across LFP electrodes prepared and cycled with liquid electrolyte. This can be understood because the high ion conductivity of liquid electrolyte leads to almost uniform electrodes during electrochemical cycling. Third, it was recently found that LFP electrode goes through the particle-by-particle (de)lithiation pathway [32] . Our results clearly show that such phase migration starts in the region adjacent to the current collector. The intriguing contrast of in situ sXAS between NMC and LFP electrodes is another substantial observation of the charge dynamics in battery electrodes. The different types of phase transformations have important roles here. The solid solution and the dominating two-phase transformation in NMC and LFP, respectively, are evident in both sXAS ( Supplementary Fig. S6 ) and electrochemical data ( Fig. 2c and Fig. 3c ) [21] , [22] . For solid-solution type transitions in NMC, the monotonic correlation between SOC and potential ( Fig. 2c ) provides the intrinsic driving force for interparticle charge transportation, which tends to form uniform electrodes. However for LFP, the potential plateaus over a large range of SOC ( Fig. 3c ) clearly shows that such a driving force is completely lost. Additionally, as discussed above, the open-circuit relaxation is driven by ion diffusion, thus strongly depending on the ion conductivity. This effect is amplified by the polymer electrolyte, which typically has low conductivity. It is known that the ion conductivity in PEO electrolyte is determined by the local segmental motion of the polymer [33] . Such motion is restrained when PEO is absorbed on the active material surface, leading to decreased ion conductivity. As tested by the BET technique, the surface area of LFP (12.823 m 2 g −1 ) is 75 times larger than that of NMC (0.171 m 2 g −1 ). Moreover, the PEO electrolyte matrix forms their own micron-sized domains between large NMC secondary particles ( Fig. 1d ) [25] . However in LFP electrodes, the PEO is superficially distributed on the surface of the nanoparticles ( Fig. 1e ). Therefore, the ion conductivity of PEO could suffer more surface retardation effect in LFP than in NMC. The decreased ion conductivity of PEO electrolyte on the active material surface lengthens the relaxation time, which is dramatic in LFP electrodes. Finally, we would emphasize that, during electrochemical cycling, the phase transformation starts from the region close to the current collector ( Fig. 5 ). This indicates that electron transportation is the determining factor during the charge process. It is known that electronic conductivity of LFP materials is intrinsically low, which contributes to this phenomenon. Still, it is surprising that such effect manifests even with 5% loading of conductive additive (see Methods). During the relaxation process, the electric circuit is open and the ion conductivity becomes more important. Therefore, the open-circuit relaxation time strongly depends on the temperature ( Fig. 4a ) and electrolyte concentration ( Supplementary Fig. S5 ). The crossover of the determining factors—that is, electron conductivity during cycling and ion conductivity during open-circuit relaxation—leads to the complicated experimental observations. In summary, developments of in situ and operando sXAS tools empower us to discover the distinct charge dynamics in NMC and LFP cathodes. sXAS of NMC electrodes responds immediately to electrochemical operations and quantitatively follows the overall SOC, indicating a uniform SOC across the electrodes. On the contrary, strong relaxation and SOC gradient effects are found in LFP electrodes. The data reveal that phase transformation in our LFP electrodes starts from the region adjacent to current collectors. The electrodes take hours of relaxation time to reach a uniform SOC distribution. The cooperation of the charge conductivity, the phase transformation mechanism and the mesoscale morphology leads to the observed contrast on charge dynamics in NMC and LFP electrodes. For LFP, electron transportation is the determining factor during electrochemical cycling; however, the open-circuit relaxation time depends on ion conductivity. The driving force of the relaxation in LFP cathode under open-circuit condition remains a mystery, which calls for theoretical simulations and further experimental studies. In situ X-ray studies of the LIBs at different cycling rates and with different electrolytes will help further clarifying microscopic mechanisms of the charge dynamics. This comparative study demonstrates the power of in situ sXAS on revealing the charge dynamics in battery electrodes. The application of the developed in situ sXAS could be extended for studying other electrode systems as well as solid-state electrolytes. In situ and ex situ battery cell preparation The cells are composed of a lithium foil anode, a solid polymer electrolyte and an NMC (or LFP) composite cathode. All the materials are rigorously dried, stored and handled in the glove boxes filled with argon (<1 p.p.m. H 2 O, O 2 ). To prepare the in situ electrodes, aluminium current collectors are first drilled with a computerized, high-precision and high-power laser system (Oxford Laser Industrial System). In order to maintain the standard electrochemical operation, we extensively explored and optimized configurations of different hole shapes (round or square), sizes (50–200 μm), distances (100–200 μm) and patterns. The reported in situ results reported here are collected with round detection holes of 50 μm diameter and 100 μm distance. NMC (Applied Materials, average secondary particle size ca . 6 μm formed by small particles of 200–300 nm) and LFP (Hydro Québec, average particle size ca . 300 nm) are used as active materials. They are mixed with AB conductive additive, PEO binder and LiTFSI salt (molar ratio of Li/O=1/10) in acetonitrile to make slurry. After evaporation of acetonitrile, the composite cathode is also dried at 70 °C under vacuum overnight. Three different cathode electrodes are made ( Supplementary Table S1 ): NMC: binder (PEO-LiTFSI): AB=70:25:5; LFP: binder (PEO-LiTFSI): AB=70:25:5 and LFP: binder (PEO-LiTFSI): AB=54:39:7, with average thickness of about 23, 27 and 29 μm, respectively. To prepare the PEO:LiTFSI solid electrolyte, PEO (Aldrich, molecular weight M W ≈1,000,000 g mol −1 ) and LiTFSI (Aldrich) are dissolved in acetonitrile (Aldrich) with a molar ratio of Li/O=1/10. Benzophenone (Aldrich) as the photoinitiator is added (10% by weight with PEO) latter. The clear polymer solutions are cast in glass O-ring molds on a polytetrafluoroethylene plate, and PEO-LiTFSI solid ionic conducting membranes are obtained ( ca . 300 μm thickness) after evaporation of the acetonitrile solvent. Finally, the PEO-LiTFSI membranes are illuminated with ultraviolet (UV) light in a portable UV light-curing system (Uvitron International, PORTA-RAY 400R system) to properly crosslink PEO and are heated at 70 °C under vacuum overnight for use. The cells for in situ test are assembled inside the argon-filled glove box on a specially designed sample holder and then transferred to ultrahigh vacuum via a kit for sXAS measurement. Cathode electrodes for ex situ sXAS are prepared by loading the same slurry on normal Al foils to make pouch cells, cycled in an oven at 70 °C. The cathodes are peeled off immediately after the cycling inside a glove box and transferred to ultrahigh vacuum without air exposure for ex situ s XAS. Electrochemical cycling All seven cells reported here were cycled at constant current at 348 K to ensure the optimized ion conductivity in solid PEO electrolyte. The current is calculated so that the theoretical time for full charge/discharge is 5 h, that is, C/5 rate. The voltage range was 2.8–4.2 V versus Li/Li + for NMC and 2.8–4.0 V versus Li/Li + for LFP. Electron microscope and electrode morphology We performed SEM and energy dispersive X-ray spectroscopy to confirm that the cathode materials are confined inside the holes with negligible spill ( Fig. 1d,e , Supplementary Fig. S1 ). The surface morphology of electrodes in small holes was imaged with a JEOL JSM-7500F field-emission SEM, viewing from the top. The surface chemistry was mapped with an energy dispersive X-ray analyser from Thermo Scientific Analysis. Specific surfaces of NMC and LFP materials are determined using the TriStar II analyzer from Micromeritics Instrument Corporation through the BET method. The optical micrograph of the electrode was taken with a Nikon Eclipse LV100 microscope. Soft X-ray spectroscopy The sXAS was performed at the undulator Beamline 8.0.1 of the Advanced Light Source (ALS) at Lawrence Berkeley National Laboratory (LBNL). The beamline is equipped with a spherical grating monochromator and supplies linearly polarized soft X-ray with resolving power up to 6,000. sXAS TFY signals are collected simultaneously with the electrochemical cycling by using a channeltron electron multiplier. The TEY spectra were obtained by measuring the photoemission current, which required stopping of the electrochemical cycling intermittently. The energy resolution of the sXAS spectra is better than 0.15 eV without considering core-hole lifetime broadening effect. All the spectra are normalized to the photon flux of incident beam monitored by the photocurrent from a clean gold mesh. In order to avoid radiation-damage issue for in situ sXAS measurements, both the incident beam brightness and data collection time are reduced. The X-ray beam is defocused with a bendable soft X-ray-refocusing mirror system to a large beam size of about 2 mm × 5 mm. The defocused beam is truncated with X-ray baffles along both horizontal and vertical directions and positioned on the detection-hole area of the in situ battery cells ( Fig. 1 ). The successful cycling of the battery cells with real-time response in sXAS data ( Fig. 2 ) testifies that the reduction on X-ray brightness efficiently avoids irradiation effect in the sensitive compounds, such as the organic electrolyte and binder. How to cite this article: Liu, X. et al. Distinct charge dynamics in battery electrodes revealed by in situ and operando soft X-ray spectroscopy. Nat. Commun. 4:2568 doi: 10.1038/ncomms3568 (2013).